Honokiol blocks and reverses cardiac hypertrophy in mice by activating mitochondrial Sirt3 Honokiol (HKL) is a natural biphenolic compound derived from the bark of magnolia trees with anti-inflammatory, anti-oxidative, anti-tumour and neuroprotective properties. Here we show that HKL blocks agonist-induced and pressure overload-mediated, cardiac hypertrophic responses, and ameliorates pre-existing cardiac hypertrophy, in mice. Our data suggest that the anti-hypertrophic effects of HKL depend on activation of the deacetylase Sirt3. We demonstrate that HKL is present in mitochondria, enhances Sirt3 expression nearly twofold and suggest that HKL may bind to Sirt3 to further increase its activity. Increased Sirt3 activity is associated with reduced acetylation of mitochondrial Sirt3 substrates, MnSOD and oligomycin-sensitivity conferring protein (OSCP). HKL-treatment increases mitochondrial rate of oxygen consumption and reduces ROS synthesis in wild type, but not in Sirt3-KO cells. Moreover, HKL-treatment blocks cardiac fibroblast proliferation and differentiation to myofibroblasts in a Sirt3-dependent manner. These results suggest that HKL is a pharmacological activator of Sirt3 capable of blocking, and even reversing, the cardiac hypertrophic response. Cardiac hypertrophy is a physiologic or pathologic state of the heart that occurs in response to a variety of intrinsic or extrinsic stimuli. Fully differentiated cardiac myocytes achieve this by increase in size, enhanced protein synthesis and increased sarcomere organization, in association with reactivation of the fetal gene programme. Even though this could be a compensatory response initially to normalize increased wall tension of the ventricles, sustained increase in hypertrophy leads to ventricular dilatation and heart failure. At the molecular level cardiac hypertrophy is a consequence of imbalance between the activities of pro- and anti-hypertrophic molecules. We have previously demonstrated that Sirt3 is one of the anti-hypertrophic molecules whose deficiency causes development of hypertrophy, whereas cardiac specific overexpression of Sirt3 blocks the hypertrophic response [1] . Sirt3 is a class III HDAC predominantly located in mitochondria, which also harbours two other sirtuins, SIRT4 and SIRT5 (ref. 2 ). All these sirtuins impart post-translational modifications in target proteins to regulate their function. Among them, Sirt3 is the only one which exhibits robust deacetylase activity [3] , [4] . A recent study showed that >65% of the total mitochondrial proteins are acetylated, and Sirt3 is the primary deacetylase involved in their deacetylation [5] . Sirt3-knockout mice do not show any noticeable phenotype at birth, and because of this reason it is believed that Sirt3 does not play a role in the embryonic development, but rather it fine tunes the activity of mitochondrial substrates by lysine deacetylation to protect cells from stress [6] . The substrates of Sirt3 are very diverse and include enzymes, which serve unique and critical functions regulating metabolism, cell survival and longevity [7] , [8] , [9] . Sirt3 deficiency manifests in reduced cellular ATP and increased ROS levels. Sirt3-knockout mice have 50% less ATP levels than their wild-type littermates, and are prone to develop cardiac hypertrophy at an early age [1] , [3] . These mice also develop age-related hearing loss and are susceptible to develop cancer [10] , [11] . More than 90% of the Sirt3-KO mice develop hepatocellular carcinoma, and show characteristics of metabolic syndrome when fed with high-fat diet [10] . Similarly, Sirt3 levels were reduced in many experimental models of cancer, diabetes mellitus and heart failure [1] , [9] , [12] . Correspondingly, nearly 40% reduced Sirt3 levels were found in older patients (60 plus years) with sedentary life style. After endurance exercise Sirt3 levels were increased significantly and they were found to be associated with health benefits to patients [13] . In population studies, increased Sirt3 level due to polymorphism in the gene promoter was linked to extended lifespan of humans, whereas another polymorphism in the Sirt3 gene led to decreased enzymatic activity of Sirt3, and was found to be associated with metabolic syndrome in humans, thus implicating a role of Sirt3 in regulating human ageing [14] , [15] . From these studies it is apparent that increasing intracellular levels of Sirt3 would be a strategy to ameliorate development of many diseases and health deficiencies associated with ageing. So far, calorie restriction is considered as the most robust intervention to improve health and longevity of animals [16] . Accordingly, calorie restriction and endurance exercise are the only available approaches to increase intracellular levels of Sirt3 (refs 11 , 17 , 18 , 19 ). Calorie restriction is associated with reduced mitochondrial protein acetylation and improved cellular functions [5] . Since calorie restriction is infeasible for every patient, discovery of a pharmacological activator of Sirt3 is highly desirable for the treatment of many diseases associated with Sirt3 deficiency. To our knowledge no pharmacological activators of Sirt3 has been reported so far. Resveratrol, a polyphenolic compound, found in grapes and wine was shown to activate SIRT1 and SIRT5, while having no effect on Sirt3 (refs 20 , 21 ). HKL [2-(4-hydroxy-3-prop-2-enyl-phenyl)-4-prop-2-enyl-phenol] is a small molecular weight natural biphenolic compound derived from the bark of magnolia trees, which is used in a traditional Asian medicinal system [22] . Pharmaceutically, it has analgesic, anti-inflammatory, anti-oxidative, anti-tumour and neuroprotective properties [22] , [23] , [24] , [25] . Oral administration of HKL prevents age-related learning and memory impairment and neuronal deficits in senescence-accelerated mice [26] . In rats, HKL ameliorates cerebral infarction resulting from ischaemia reperfusion injury, via inhibition of neutrophil infiltration and reactive oxygen species (ROS) production [27] . With regard to cancer, HKL not only induces apoptosis in a variety of tumours, but also reverses TGFβ and TNFα-induced epithelial–mesenchymal transition in spontaneously immortalized non-tumorigenic human mammary epithelial cells [22] . All these findings imply that HKL is a bioactive compound possessing cytoprotective capabilities. In this study, we report that the biphenolic compound HKL upregulates Sirt3 levels both in cells and animals. We also demonstrate that HKL-mediated upregulation of Sirt3 blocks the cardiac hypertrophic response in vitro as well as in vivo . To the best of our knowledge this is the first report describing a pharmacological activator of Sirt3. HKL increases Sirt3 levels and its activity Sirt3 has been recognized as a major deacetylase of mitochondria. To identify an activator of Sirt3, we analysed effects of different pharmacological compounds on the acetylation status of mitochondrial proteins. In our search we found that treatment of cardiomyocytes with honokiol (HKL) substantially reduced mitochondrial protein acetylation in a dose-dependent manner, but not the derivative 2,4′dihydroxybiphenyl (DHBP), which served as a negative control ( Fig. 1a , Supplementary Fig. 1 ). These results suggested that HKL might have potential to activate Sirt3. We then asked if HKL can reduce mitochondrial acetylation in a time-dependent manner. Cardiomyocytes were treated with 10 μM HKL and the mitochondrial protein acetylation was determined at indicated time points. The results showed that HKL can reduce mitochondrial acetylation with increasing time, again indicative of increased Sirt3 activity ( Fig. 1b ). We then asked whether HKL treatment can increase cellular levels of Sirt3. Since we found optimum Sirt3 activation at 24 h, we treated cardiomyocytes with 5 or 10 μM HKL for 24 h, and analysed Sirt3 levels by immunoblotting. Both doses of HKL increased Sirt3 levels by nearly twofold ( Fig. 1c,d ). To test whether increased Sirt3 levels were associated with its increased activity, we analysed acetylation status of the two Sirt3 substrates, MnSOD and OSCP (oligomycin-sensitivity conferring protein), using antibodies that specifically detect MnSOD acetylation at K-122 and OSCP acetylation at K-139. Deacetylation of MnSOD at K-122 by Sirt3 has been shown to increase its activity [28] . Consistent with increased Sirt3 levels, we observed increased activity of Sirt3 as revealed by reduced acetylation of MnSOD and OSCP following HKL treatment ( Fig. 1c ). Quantification of data showed that HKL treatment has far more effect on activity of Sirt3 than that can be correlated with its increased protein levels ( Fig. 1e,f ). In this assay we also measured the effect of HKL on SIRT1 and Nampt; however, we found no appreciable effects ( Fig. 1c ). Collectively, these data indicated that HKL is capable of activating mitochondrial Sirt3. 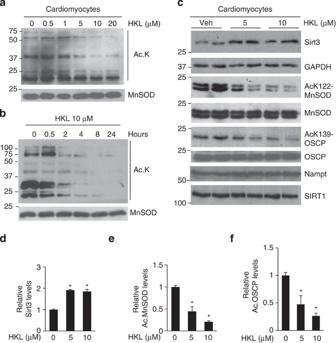Figure 1: HKL activates Sirt3 and deacetylates mitochondrial proteins. (a) Primary cultures of neonatal rat cardiomyocytes were treated with different doses of HKL as indicated. Mitochondrial lysate was prepared and analysed for lysine-acetylation using an anti-acetyl lysine antibody (Ac-K). Total MnSOD level served as a loading control. (b) Primary cultures of neonatal rat cardiomyocytes were treated with 10 μM HKL at different time points as indicated. Mitochondrial lysate was prepared and analysed for lysine-acetylation using an anti-acetyl lysine antibody. (c) Primary cultures of cardiomyocytes were treated with 5 and 10 μM HKL for 24 h. Cell lysate was analysed by western blotting with indicated antibodies. (d–f) Quantification of relative Sirt3, acetylated (Ac) MnSOD and acetylated OSCP levels in cardiomyocytes treated with HKL. Values are average of four independent experiments, mean±s.e. *P<0.05; Studentst-test. Figure 1: HKL activates Sirt3 and deacetylates mitochondrial proteins. ( a ) Primary cultures of neonatal rat cardiomyocytes were treated with different doses of HKL as indicated. Mitochondrial lysate was prepared and analysed for lysine-acetylation using an anti-acetyl lysine antibody (Ac-K). Total MnSOD level served as a loading control. ( b ) Primary cultures of neonatal rat cardiomyocytes were treated with 10 μM HKL at different time points as indicated. Mitochondrial lysate was prepared and analysed for lysine-acetylation using an anti-acetyl lysine antibody. ( c ) Primary cultures of cardiomyocytes were treated with 5 and 10 μM HKL for 24 h. Cell lysate was analysed by western blotting with indicated antibodies. ( d – f ) Quantification of relative Sirt3, acetylated (Ac) MnSOD and acetylated OSCP levels in cardiomyocytes treated with HKL. Values are average of four independent experiments, mean±s.e. * P <0.05; Students t -test. Full size image HKL blocks hypertrophic response of cardiomyocytes in vitro On the basis of previous reports showing that Sirt3 protects cardiomyocytes from hypertrophic stimuli, we asked whether HKL can also protect cardiomyocytes from developing hypertrophy [1] . To this end, cardiomyocytes were treated with a hypertrophic agonist phenylephrine (PE) in the presence or absence of HKL. After 48 h of treatment cells were harvested and mitochondrial acetylation was analysed by western blotting. PE-treated cardiomyocytes showed increased acetylation, whereas this acetylation was reduced in HKL-treated cardiomyocytes ( Fig. 2a ). Consistent with this we also observed increased levels of Sirt3 in HKL-treated samples ( Fig. 2a ). Hypertrophy of cardiomyocytes was evaluated by measuring incorporation of [ 3 H]-leucine into total cellular proteins, a marker of hypertrophy. HKL treatment dose dependently attenuated PE-induced [ 3 H]-leucine incorporation into total cellular proteins of cardiomyocytes ( Fig. 2b ). Hypertrophic stimuli are known to cause translocation of NFAT into the nucleus, resulting in activation of hypertrophic gene programme [29] . To investigate whether HKL can block agonist-induced NFAT activation, cardiomyocytes were infected with an adenovirus vector expressing NFAT promoter-luciferase reporter gene, and treated with PE in the presence or absence of HKL. HKL treatment abolished the PE-induced activation of the NFAT-reporter gene ( Fig. 2c ). These results were also confirmed by analysing nuclear localization of NFAT. PE-treated cardiomyocytes showed increased NFAT levels in the nuclear extract, which was not seen when cells were treated with HKL ( Fig. 2d ). HKL treatment also blocked the PE-mediated increase of cardiomyocyte size and ANF release (red) from the nuclei, other hallmarks of hypertrophy ( Fig. 2e,f ). Similarly, HKL treatment also blocked the hypertrophic response of cardiomyocytes to another agonist, angiotensin-II (Ang-II) ( Supplementary Fig. 2 ). These results thus indicated that HKL is capable of blocking the cardiac hypertrophic response in vitro . 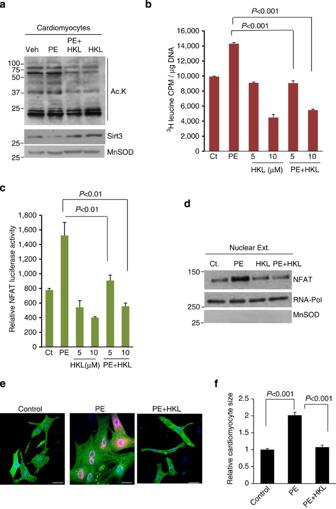Figure 2: HKL blocks induction of cardiac hypertrophic responsein vitro. (a) Primary cultures of cardiomyocytes were treated with 20 μM phenylephrine (PE) in the presence or absence of 10 μM HKL. Forty-eight hours after treatment, cells were harvested and mitochondrial lysate analysed by western blotting with use of indicated antibodies. (b) Cultures of cardiomyocytes were labelled with [3H]-leucine and then treated with PE (20 μM) in the presence or absence of 5 or 10 μM HKL. Twenty hours after treatment, cells were harvested and incorporation of [3H]-leucine into total cellular proteins was measured. Mean±s.e. values are average of three independent experiments; Student’st-test. (c) Cardiomyocytes were infected with a NFAT-responsive luciferase reporter adenovirus vector. Twelve hours after infection cells were treated with PE in the presence or absence of HKL for 8 h. HKL treatment was given 2 h before PE treatment. The luciferase activity assay was performed using an activity assay kit from Promega, as per the manufacturer’s protocol. Mean±s.e. values are average of three independent experiments; Student’st-test. (d) Cardiomyocytes were treated same as in panel ‘a’. Thereafter, nuclear lysate was prepared and analysed by western blotting with use of indicated antibodies. (e) Cardiomyocytes were treated with PE in the presence or absence of 10 μM HKL. Cardiomyocytes were identified by α-actinin staining (green) and the release of ANF from nuclei was determined by staining cells with an anti-ANF antibody (red). DAPI stain was used to mark the position of nuclei. Scale bars, 25 μm. (f) Cardiomyocyte size of α-actinin positive cells was quantified by use of Image J software. Values are expressed as fold change with respect to untreated control. Mean±s.e. values are average of three independent experiments; Student’st-test. Figure 2: HKL blocks induction of cardiac hypertrophic response in vitro . ( a ) Primary cultures of cardiomyocytes were treated with 20 μM phenylephrine (PE) in the presence or absence of 10 μM HKL. Forty-eight hours after treatment, cells were harvested and mitochondrial lysate analysed by western blotting with use of indicated antibodies. ( b ) Cultures of cardiomyocytes were labelled with [ 3 H]-leucine and then treated with PE (20 μM) in the presence or absence of 5 or 10 μM HKL. Twenty hours after treatment, cells were harvested and incorporation of [ 3 H]-leucine into total cellular proteins was measured. Mean±s.e. values are average of three independent experiments; Student’s t -test. ( c ) Cardiomyocytes were infected with a NFAT-responsive luciferase reporter adenovirus vector. Twelve hours after infection cells were treated with PE in the presence or absence of HKL for 8 h. HKL treatment was given 2 h before PE treatment. The luciferase activity assay was performed using an activity assay kit from Promega, as per the manufacturer’s protocol. Mean±s.e. values are average of three independent experiments; Student’s t -test. ( d ) Cardiomyocytes were treated same as in panel ‘ a ’. Thereafter, nuclear lysate was prepared and analysed by western blotting with use of indicated antibodies. ( e ) Cardiomyocytes were treated with PE in the presence or absence of 10 μM HKL. Cardiomyocytes were identified by α-actinin staining (green) and the release of ANF from nuclei was determined by staining cells with an anti-ANF antibody (red). DAPI stain was used to mark the position of nuclei. Scale bars, 25 μm. ( f ) Cardiomyocyte size of α-actinin positive cells was quantified by use of Image J software. Values are expressed as fold change with respect to untreated control. Mean±s.e. values are average of three independent experiments; Student’s t -test. Full size image HKL protects mice from developing cardiac hypertrophy We next tested the ability of HKL to block development of cardiac hypertrophy in vivo . Mice were subjected to TAC for 28 days. Second day after surgery, HKL treatment was started (0.2 mg kg −1 day −1 ) and it was maintained throughout the course of study. TAC induction in control mice resulted in 25% cardiac hypertrophy as estimated by heart weight to body weight ratio (HW/BW) ( Fig. 3a ). This was associated with increased ventricular wall thickness and activation of the fetal gene programme (collagen, β-MHC and ANF). These changes were markedly reduced in HKL-treated mice ( Fig. 3b , Supplementary Fig. 3a ). HKL treatment also reduced TAC-induced accumulation of fibrosis in the interstitial space and increase in cardiomyocyte size as revealed by Masson’s trichrome staining and WGA staining, respectively ( Fig. 3c–e ). We also tested Sirt3 levels and its activity in mice underwent to TAC. Sirt3 levels were markedly reduced in mice subjected to TAC, but were maintained to control levels in HKL-treated mice ( Fig. 3f ). This increase in Sirt3 levels also correlated with the acetylation status of MnSOD. MnSOD was hyperacetylated in mice subjected to TAC, whereas HKL treatment restored it to control levels ( Fig. 3f , Supplementary Fig. 3b ). These results suggested that HKL is also capable of activating Sirt3 and blocking the cardiac hypertrophic response in vivo . 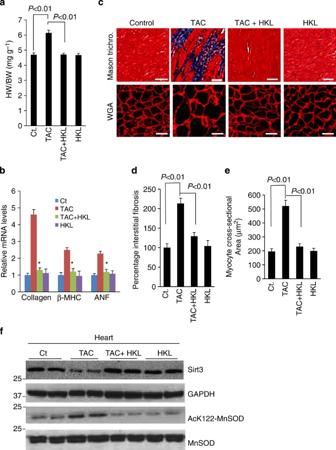Figure 3: HKL blocks induction of cardiac hypertrophic responsein vivo. (a) Heart weight body weight (HW/BW) ratio of control (Ct), TAC (transverse aortic constriction) and TAC mice treated with HKL, mean±s.e.,n=8–10 mice. (b) Expression levels of collagen-1, β-MHC and ANF mRNA in different groups of mice, mean±s.e.,n=8–10 mice, *P<0.01 compared with TAC alone. (c) Top panel, sections of hearts stained with Masson’s trichrome to detect fibrosis (blue); scale bars, 20 μm; bottom panel, heart sections stained with wheat germ agglutinin (WGA) to demarcate cell boundaries, scale bars, 10 μm. (d,e) Quantification of cardiac fibrosis and myocyte cross-sectional area in different groups of mice. Mean±s.e.,n=5 mice. For the panelsa,b,dande, ANOVA was applied to calculate thePvalue. (f) Heart lysate of different groups of mice was subjected to immunoblotting using indicated antibodies. Results of two mice in each group are shown. Figure 3: HKL blocks induction of cardiac hypertrophic response in vivo . ( a ) Heart weight body weight (HW/BW) ratio of control (Ct), TAC (transverse aortic constriction) and TAC mice treated with HKL, mean±s.e., n =8–10 mice. ( b ) Expression levels of collagen-1, β-MHC and ANF mRNA in different groups of mice, mean±s.e., n =8–10 mice, * P <0.01 compared with TAC alone. ( c ) Top panel, sections of hearts stained with Masson’s trichrome to detect fibrosis (blue); scale bars, 20 μm; bottom panel, heart sections stained with wheat germ agglutinin (WGA) to demarcate cell boundaries, scale bars, 10 μm. ( d , e ) Quantification of cardiac fibrosis and myocyte cross-sectional area in different groups of mice. Mean±s.e., n =5 mice. For the panels a , b , d and e , ANOVA was applied to calculate the P value. ( f ) Heart lysate of different groups of mice was subjected to immunoblotting using indicated antibodies. Results of two mice in each group are shown. Full size image HKL attenuates pre-established cardiac hypertrophy in mice Knowing that HKL possess anti-hypertrophic activity, we next investigated whether HKL can reverse pre-existing (post-banding) cardiac hypertrophy, which is a more clinically relevant situation. Mice were subjected to aortic banding to develop hypertrophy for 4 months. Once the hypertrophy was established, they were treated with HKL for 28 days. As shown in Fig. 4a , HKL treatment significantly reduced the HW/BW ratio in mice subjected to TAC. Consistent with this, HKL treatment also decreased the ventricular wall thickness and improved the fractional shortening following TAC, compared with untreated mice ( Fig. 4b,c ). In addition, HKL treatment significantly reduced the accumulation of interstitial fibrosis and activation of the fetal gene programme ( Fig. 4d,e,f ). We then analysed the effect of HKL on the signalling programme that is known to be activated during hypertrophy. Increased Akt activation is known to induce cardiac hypertrophy in response to variety of stresses [30] . We therefore examined the role of HKL in regulating the Akt signalling. Increased phosphorylation of Akt was observed in banded mice, and HKL treatment helped to maintain it to control levels. Consistent with Akt, ERK1/2 was also activated in TAC mice, and HKL was capable of blocking its activation. In accordance with this, there was increased phosphorylation of S6 ribosomal protein in TAC mice, whereas HKL treatment restored it back to normal levels, thus suggesting that HKL negatively regulated the cardiac hypertrophic response by controlling the Akt signalling pathway ( Fig. 4g ). Together, these data indicated that HKL treatment is capable of blocking both the induction and progression of cardiac hypertrophy. 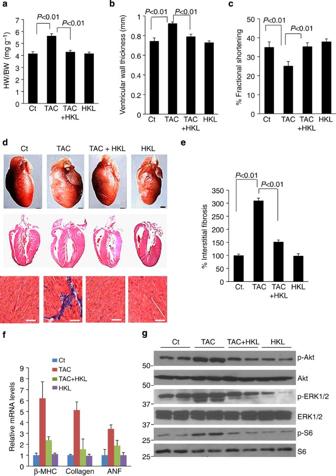Figure 4: HKL attenuates pre-established cardiac hypertrophy in mice. (a) Mice were subjected to TAC for 4 months and then treated with HKL for 28 days. Bar diagram shows HW/BW ratio of control, TAC, TAC mice treated with HKL and HKL alone, mean±s.e.,n=5–8 mice; ANOVA. (b,c) Echocardiographic measurements of ejection fraction and fractional shortening in control, TAC, TAC treated with HKL and HKL alone mice. For panelsa–c, mean±s.e.,n=5–8 mice; ANOVA was applied to calculate thePvalue. (d) Top panel, whole heart of control, TAC and TAC treated with HKL and HKL alone mice; scale bars, 1 mm; middle panel, H & E-stained sections of whole hearts of different groups of mice; scale bars, 1 mm; bottom panel, sections of hearts stained with Masson’s trichrome to detect fibrosis (blue); scale bars, 20 μm. (e) Quantification of cardiac fibrosis in different groups of mice, mean±s.e.,n=5–8 mice; ANOVA was applied to calculate thePvalue. (f) β-myosin heavy chain(MHC), collagen-1 and ANF mRNA levels in the heart samples of control, TAC alone and TAC plus HKL and HKL alone treated mice. (g) Heart lysates of different groups of mice were subjected to immunoblotting with antibodies as indicated. Results are shown for two animals of each group. Figure 4: HKL attenuates pre-established cardiac hypertrophy in mice. ( a ) Mice were subjected to TAC for 4 months and then treated with HKL for 28 days. Bar diagram shows HW/BW ratio of control, TAC, TAC mice treated with HKL and HKL alone, mean±s.e., n =5–8 mice; ANOVA. ( b , c ) Echocardiographic measurements of ejection fraction and fractional shortening in control, TAC, TAC treated with HKL and HKL alone mice. For panels a – c , mean±s.e., n =5–8 mice; ANOVA was applied to calculate the P value. ( d ) Top panel, whole heart of control, TAC and TAC treated with HKL and HKL alone mice; scale bars, 1 mm; middle panel, H & E-stained sections of whole hearts of different groups of mice; scale bars, 1 mm; bottom panel, sections of hearts stained with Masson’s trichrome to detect fibrosis ( blue ); scale bars, 20 μm. ( e ) Quantification of cardiac fibrosis in different groups of mice, mean±s.e., n =5–8 mice; ANOVA was applied to calculate the P value. ( f ) β-myosin heavy chain (MHC) , collagen-1 and ANF mRNA levels in the heart samples of control, TAC alone and TAC plus HKL and HKL alone treated mice. ( g ) Heart lysates of different groups of mice were subjected to immunoblotting with antibodies as indicated. Results are shown for two animals of each group. Full size image Sirt3 mediates anti-hypertrophic activity of HKL To gain evidence that anti-hypertrophic effects of HKL were mediated via activation of Sirt3, we measured its effect in Sirt3-deficient hearts. Sirt3-KO mice along with their wild-type controls were chronically infused with the hypertrophic agonist isoproterenol (ISO) (Sirt3-KO mice did not tolerate TAC), either alone or together with HKL. The results showed that both HKL-treated and untreated Sirt3-KO mice had a significantly increased hypertrophic response, as determined by HW/BW ratio, interstitial fibrosis and expression of collagen-1 mRNA levels, thus suggesting that HKL was unable to block hypertrophic response of Sirt3-KO heart, whereas it was capable of doing so in wild-type hearts ( Fig. 5a–c , Supplementary Fig. 4 ). We also found that chronic isoproterenol treatment reduced Sirt3 levels and increased MnSOD acetylation, which was reversed back to control levels by HKL treatment in wild-type, but not in Sirt3-KO mice ( Fig. 5d ). These data thus demonstrated involvement of Sirt3-mediated signalling in anti-hypertrophic effects of HKL. 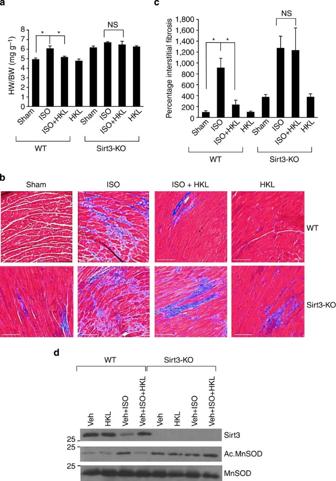Figure 5: HKL treatment blocks cardiac hypertrophy of wild type, but not Sirt3-KO mice. (a) Heart weight body weight ratio of control (sham), isoproterenol (ISO) or ISO plus HKL treated wild-type (WT) and Sirt3-KO mice. Mean±s.e.,n=5–8 mice. *P<0.05, NS, not significant; ANOVA. (b) Heartsections stained with Masson’s trichrome to detect fibrosis(blue); scale, 20 μm. (c) Quantification of cardiac fibrosis in different groups of mice. Mean±s.e.,n=5 mice. *P<0.001, NS, not significant; ANOVA. (d) Heart lysates analysed by immunoblotting for the indicated antibodies. Figure 5: HKL treatment blocks cardiac hypertrophy of wild type, but not Sirt3-KO mice. ( a ) Heart weight body weight ratio of control (sham), isoproterenol (ISO) or ISO plus HKL treated wild-type (WT) and Sirt3-KO mice. Mean±s.e., n =5–8 mice. * P <0.05, NS, not significant; ANOVA. ( b ) Heart s ections stained with Masson’s trichrome to detect fibrosis (blue ); scale, 20 μm. ( c ) Quantification of cardiac fibrosis in different groups of mice. Mean±s.e., n =5 mice. * P <0.001, NS, not significant; ANOVA. ( d ) Heart lysates analysed by immunoblotting for the indicated antibodies. Full size image HKL blocks proliferation and differentiation of cardiac fibroblasts Interstitial fibrosis is one of the hallmarks of maladaptive cardiac hypertrophy. As HKL treatment reduced interstitial fibrosis in the TAC and isoproterenol models, we asked whether HKL can block proliferation and differentiation of cardiac fibroblasts to myofibroblasts, an essential marker of fibrosis. We measured fibroblasts proliferation by analysing BrdU incorporation into cellular DNA by FACS analysis. HKL treatment dose dependently reduced the proportion of S-phase cells, while increasing the proportion of G0-G1 cells, suggesting that HKL was capable of blocking cardiac fibroblasts proliferation in the G0–G1 phase ( Fig. 6a,b ). We next determined the effect of HKL on transformation of cardiac fibroblasts into myofibroblasts, by using smooth muscle alpha actin (SMA), fibronectin and collagen-1 as critical determinants of myofibroblast differentiation. Stimulation of fibroblasts with the pro-fibrotic agent Ang-II resulted in marked increase in stress fibre formation and expression of SMA and fibronectin. These changes were blocked when cells were treated with HKL, suggesting that HKL attenuated fibroblasts differentiation into myofibroblasts ( Fig. 6c,d and Supplementary Fig. 5 ). We also determined whether inhibition of cardiac fibroblasts differentiation is mediated through Sirt3. To address this issue, adult cardiac fibroblasts from wild type and Sirt3-KO mice were treated with Ang-II with or without HKL. HKL was capable of blocking Ang-induced differentiation of wild-type fibroblasts, whereas Sirt3-KO fibroblasts spontaneously differentiated into myofibroblasts, and HKL had no effect on this transformation, as indicated by expression of collagen-1 and SMA staining, suggesting that HKL inhibits fibroblast differentiation via activation of Sirt3 ( Fig. 7a–c , Supplementary Fig. 6 ). These results again demonstrated the involvement of Sirt3 for antifibrotic effects of HKL. 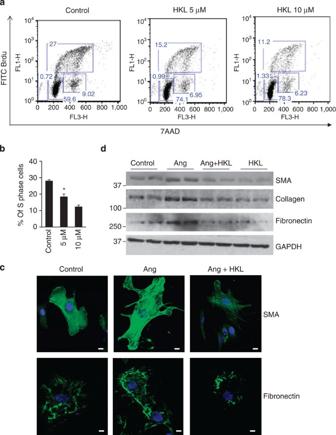Figure 6: HKL attenuates cardiac fibroblasts proliferation and differentiation into myofibroblasts. (a) Rat cardiac fibroblasts cultured in complete growth medium were treated with 5 or 10 μM HKL. Sixteen hours after HKL treatment cells were treated with BrdU (10 μM) for 2 h. Cells were harvested, stained with an anti-Brdu antibody (Y-axis) and 7AAD (X-axis) and subjected to FACS analysis. (b) Quantification of S-phase cells. Mean±s.e., values are average of three independent experiments, *P<0.05 compared with control; Studentst-test. (c) Cardiac fibroblasts were treated with 100 nM angiotensin-II (Ang) in the presence of 500 nM HKL for 72 h. Cells were immunostained for α-SMA and fibronectin; Scale 10 μm. (d) Primary cultures of cardiac fibroblasts were treated with 100 nM Ang in the presence or absence of HKL for 72 h. Cell lysates were prepared and analysed by western blotting with indicated antibodies. Results are shown for two samples in each group. Figure 6: HKL attenuates cardiac fibroblasts proliferation and differentiation into myofibroblasts. ( a ) Rat cardiac fibroblasts cultured in complete growth medium were treated with 5 or 10 μM HKL. Sixteen hours after HKL treatment cells were treated with BrdU (10 μM) for 2 h. Cells were harvested, stained with an anti-Brdu antibody (Y-axis) and 7AAD (X-axis) and subjected to FACS analysis. ( b ) Quantification of S-phase cells. Mean±s.e., values are average of three independent experiments, * P <0.05 compared with control; Students t -test. ( c ) Cardiac fibroblasts were treated with 100 nM angiotensin-II (Ang) in the presence of 500 nM HKL for 72 h. Cells were immunostained for α-SMA and fibronectin; Scale 10 μm. ( d ) Primary cultures of cardiac fibroblasts were treated with 100 nM Ang in the presence or absence of HKL for 72 h. Cell lysates were prepared and analysed by western blotting with indicated antibodies. Results are shown for two samples in each group. 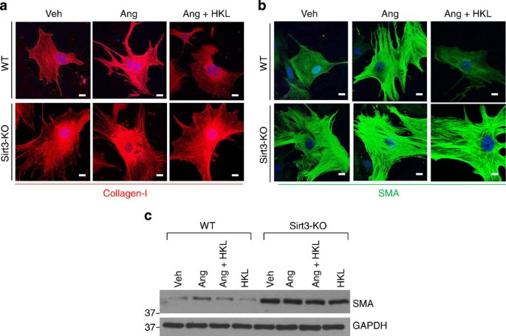Figure 7: HKL blocks differentiation of wild-type cardiac fibroblast to myofibroblasts, but not Sirt3-KO fibroblasts. (a,b) Primary cultures of mouse cardiac fibroblasts obtained from wild-type (WT) and Sirt3-KO mice were treated with 100 nM Ang in the presence or absence of HKL for 72 h. Cells were immunostained for α-SMA and collagen-1; scale bar, 10 μm. (c) Cell lysates were prepared from another set of plates and subjected to immunostaining for α-SMA. For loading control, the blot was probed with an anti-GAPDH antibody. Full size image Figure 7: HKL blocks differentiation of wild-type cardiac fibroblast to myofibroblasts, but not Sirt3-KO fibroblasts. ( a , b ) Primary cultures of mouse cardiac fibroblasts obtained from wild-type (WT) and Sirt3-KO mice were treated with 100 nM Ang in the presence or absence of HKL for 72 h. Cells were immunostained for α-SMA and collagen-1; scale bar, 10 μm. ( c ) Cell lysates were prepared from another set of plates and subjected to immunostaining for α-SMA. For loading control, the blot was probed with an anti-GAPDH antibody. Full size image HKL reduces ROS production and prevents cardiomyocyte death We have previously shown that Sirt3 protects cardiomyocytes from oxidative and genotoxic stress by reducing ROS production [7] . To get further support for the ability of HKL to activate Sirt3, we measured H 2 O 2 -induced ROS production in cardiomyocytes. Neonatal cardiomyocytes from wild type and Sirt3-KO mice were treated with H 2 O 2 in the presence or absence of HKL. As shown in Fig. 8 , HKL treatment contained H 2 O 2 -induced ROS levels in wild-type cells, but not in Sirt3-KO cells ( Fig. 8a,b ). To gather further support for these results, we also performed a cell death experiment. Consistent with our ROS results, HKL treatment helped to rescue wild-type cells from H 2 O 2 -induced cell death, but not Sirt3-KO cells, suggesting that the cytoprotective effect of HKL is mediated through activation of Sirt3 ( Fig. 8c ). To further confirm antiapoptotic activity of HKL, we also tested PARP cleavage in cardiomyocytes following H 2 O 2 treatment. As shown in Fig. 8d, H 2 O 2 treatment increased levels of cleaved PARP in cardiomyocytes, which was restored back to control levels after HKL treatment, thus supporting anti-apoptotic activity of HKL in cardiomyocytes (Fig. 8d ). To gain additional evidence that the effects of HKL are mediated via activation of mitochondrial Sirt3, we measured basal rate of oxygen consumption, a measure of mitochondrial health. Sirt3 deficiency has been shown to reduce basal mitochondrial oxygen consumption rate in many cell types, including skeletal muscle and hepatocytes [12] , [31] . We found that wild-type cardiac fibroblasts have substantially increased rate of oxygen consumption, compared with Sirt3-KO cells, and HKL treatment substantially increased oxygen consumption rate in wild-type cells, but not in Sirt3-KO cells ( Fig. 8e ). These data thus confirmed that HKL exerts its cardioprotective effects through activation of Sirt3. 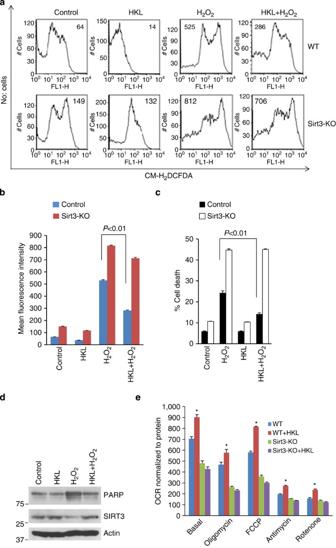Figure 8: HKL reduces ROS production and promotes cardiomyocyte survival under stress. (a) Primary cultures of cardiomyocytes obtained from wild type or Sirt3-KO mice were treated with H2O2(50 μM) in the presence or absence of HKL (10 μM) for 15 min. Cells were stained with CM-H2DCFDA. ROS levels were measured by fluorescence-activated cell sorter. (b) Quantification of the mean fluorescence intensity in different groups of cells. Values are (mean ±s.e.) average of three independent experiments; Student’st-test. (c) Primary cultures of cardiomyocytes obtained from wild-type or Sirt3-KO mice were treated with H2O2(500 μM) in the presence or absence of HKL (10 μM) for 2 h. Extend of apoptosis was measured by estimating the percentage of Annexin V-positive cells by FACS analysis. Data show quantification of cell death, mean±s.e.; values are average of three independent experiments, Studentst-test. (d) Primary cultures of cardiomyocytes were treated with H2O2(500 μM) in the presence or absence of HKL (10 μM) for 2 h. Cell lysate was analysed by western blotting with indicated antibodies. (e) Mitochondrial oxygen consumption rate (OCR) of WT and Sirt3-KO cardiac fibroblasts in response to HKL treatment, mean±s.e.; values are average of four independent experiments. *P<0.05 compared with WT untreated cells; Student’st-test. Figure 8: HKL reduces ROS production and promotes cardiomyocyte survival under stress. ( a ) Primary cultures of cardiomyocytes obtained from wild type or Sirt3-KO mice were treated with H 2 O 2 (50 μM) in the presence or absence of HKL (10 μM) for 15 min. Cells were stained with CM-H 2 DCFDA. ROS levels were measured by fluorescence-activated cell sorter. ( b ) Quantification of the mean fluorescence intensity in different groups of cells. Values are (mean ±s.e.) average of three independent experiments; Student’s t -test. ( c ) Primary cultures of cardiomyocytes obtained from wild-type or Sirt3-KO mice were treated with H 2 O 2 (500 μM) in the presence or absence of HKL (10 μM) for 2 h. Extend of apoptosis was measured by estimating the percentage of Annexin V-positive cells by FACS analysis. Data show quantification of cell death, mean±s.e. ; values are average of three independent experiments, Students t -test. ( d ) Primary cultures of cardiomyocytes were treated with H 2 O 2 (500 μM) in the presence or absence of HKL (10 μM) for 2 h. Cell lysate was analysed by western blotting with indicated antibodies. ( e ) Mitochondrial oxygen consumption rate (OCR) of WT and Sirt3-KO cardiac fibroblasts in response to HKL treatment, mean±s.e. ; values are average of four independent experiments. * P <0.05 compared with WT untreated cells; Student’s t -test. Full size image HKL directly binds to and activates Sirt3 To understand the mechanism through which HKL activates Sirt3, we asked whether HKL can directly bind to Sirt3 and enhance its enzymatic activity. Different amounts of HKL was incubated with the human Sirt3 (3 μM) and its binding to protein was measured by using fluorescence anisotropy. The results indicated reduced anisotropy values for Sirt3 with increasing amounts of HKL, suggesting a direct binding of HKL to Sirt3 ( Fig. 9a ). We next investigated whether HKL can enter into mitochondria to bind to Sirt3. Mitochondria were isolated and viability of preparation was evaluated by monitoring absorbance at 540 nm following incubation with CaCl 2 , as described in our previous studies ( Supplementary Fig. 7d ) [32] , [33] . Viable mitochondria were then incubated with 10 μM HKL for increasing time duration ranging from 0, 15, 30, 60 and 120 min. After completion of incubation time mitochondria were pelleted, washed with the incubation buffer and extracted for analysis by liquid chromatography-high-resolution mass spectrometry. The presence of HKL in mitochondria was confirmed by ion-dissociation mass-spectrometry and co-elution with the authentic standard. Increased HKL levels were observed with increasing incubation time for the isolated mitochondria, indicating HKL uptake into the matrix ( Supplementary Fig. 7a–c ). To explore whether Sirt3 activity is enhanced after binding to HKL, we tested affinity of Sirt3 for NAD. Acetylated MnSOD was incubated with decreasing concentration of NAD in the presence or absence of HKL. In this experiment reactions without NAD served as negative controls. The result of this experiment demonstrated that Sirt3 in the presence of HKL was able to deacetylate MnSOD at K122 residue at much lower concentrations of NAD, than in the absence of HKL ( Fig. 9b ). To confirm that HKL can activate Sirt3 directly in vivo , we treated cells with cycloheximide to inhibit synthesis of new Sirt3, and measured acetylation of mitochondrial proteins. We observed reduced acetylation in cycloheximide-treated cells that received HKL, suggesting that HKL can increase deacetylation of mitochondrial proteins even when no new Sirt3 is synthesized ( Fig. 9c ). These data suggest that HKL directly binds to Sirt3 and this is associated with increased enzymatic activity of Sirt3. 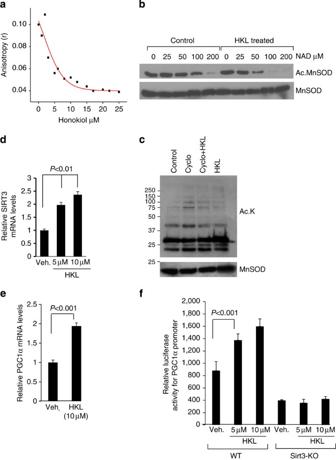Figure 9: HKL directly binds to and activates Sirt3. (a) Steady-state fluorescence anisotropy values are shown as a function of increased concentrations of HKL. The concentration of human Sirt3 was 3 μM (a representative experiment). (b) In a deacetylase buffer 0.5 μg of acetylated MnSOD was incubated with 0.5 μg of Sirt3 in the presence or absence of HKL at the indicated concentrations of NAD. Samples were analysed by immunoblotting with use of an anti-MnSOD.AcK122 antibody. Blot was stripped and probed for MnSOD for equal loading. (c) Cardiomyocytes were treated with cycloheximide (10 μM) for 1 h and then with HKL (5 μM) for next 2 h. Mitochondrial lysate was prepared and analysed by western blotting with use of indicated antibodies. (d) Sirt3 mRNA levels were measured after 6 h of treatment of cardiomyocytes with 5 and 10 μM HKL, mean±s.e.; values are average of three independent experiments; Student’st-test. (e) Cardiomyocytes were treated with 10 μM HKL and PGC1α mRNA levels were measured 6 h after treatment. Values are average of three independent experiments (mean±s.e.); Student’st-test (f) Wild-type or Sirt3-KO fibroblasts were co-transfected with a PGC1α responsive promoter/luciferase reporter plasmid. After 16 h of transfection, cells were treated with 5 or 10 μM of HKL for 8 h. Cell lysates were prepared; luciferase activity was measured and normalized to protein content, mean±s.e., Values are average of four independent experiments; Studentst-test. Figure 9: HKL directly binds to and activates Sirt3. ( a ) Steady-state fluorescence anisotropy values are shown as a function of increased concentrations of HKL. The concentration of human Sirt3 was 3 μM (a representative experiment). ( b ) In a deacetylase buffer 0.5 μg of acetylated MnSOD was incubated with 0.5 μg of Sirt3 in the presence or absence of HKL at the indicated concentrations of NAD. Samples were analysed by immunoblotting with use of an anti-MnSOD.AcK122 antibody. Blot was stripped and probed for MnSOD for equal loading. ( c ) Cardiomyocytes were treated with cycloheximide (10 μM) for 1 h and then with HKL (5 μM) for next 2 h. Mitochondrial lysate was prepared and analysed by western blotting with use of indicated antibodies. ( d ) Sirt3 mRNA levels were measured after 6 h of treatment of cardiomyocytes with 5 and 10 μM HKL, mean±s.e. ; values are average of three independent experiments; Student’s t -test. ( e ) Cardiomyocytes were treated with 10 μM HKL and PGC1α mRNA levels were measured 6 h after treatment. Values are average of three independent experiments (mean±s.e. ); Student’s t -test ( f ) Wild-type or Sirt3-KO fibroblasts were co-transfected with a PGC1α responsive promoter/luciferase reporter plasmid. After 16 h of transfection, cells were treated with 5 or 10 μM of HKL for 8 h. Cell lysates were prepared; luciferase activity was measured and normalized to protein content, mean±s.e., Values are average of four independent experiments; Students t -test. Full size image As in our initial experiments we had found increased protein levels of Sirt3 in HKL treated cells ( Fig. 1c ), we tested whether HKL can also stabilize Sirt3 protein levels. Cells were treated with cycloheximide for indicated time points in the presence or absence of HKL, and the protein levels analysed by western blotting. The presence of cycloheximide did not increase Sirt3 level in HKL-treated cells. These results thus excluded the possibility of protein stabilization as a cause of increased Sirt3 levels by HKL ( Supplementary Fig. 8 ). We then asked whether HKL can activate Sirt3 gene transcription leading to increased Sirt3 levels. Cardiomyocytes were treated with different doses of HKL (5 and 10 μM) for 6 h and then analysed for Sirt3 mRNA levels by RT-PCR analysis. HKL treatment dose dependently increased Sirt3 mRNA levels, 1.5-fold and 2-fold, respectively ( Fig. 9d ). To further confirm these results, we treated cardiomyocytes with 10 μm HKL for 3 h or 6 h and analysed for Sirt3 mRNA levels. HKL treatment increased Sirt3 levels 1.5-fold at 3 h and nearly 2-fold at 6 h, thus confirming increased Sirt3 mRNA expression by HKL ( Supplementary Fig. 9 ). The expression of Sirt3 gene is shown to be regulated by the transcription factor PGC1α, which is also sensitive to change in activity of Sirt3, thus suggesting a positive feedback mechanism controlling Sirt3 gene transcription [18] , [34] . We therefore tested whether HKL can upregulate PGC1α mRNA levels, and found twofold increase in PGC1α mRNA levels after 6 h of HKL treatment ( Fig. 9e ). We then tested the effect of HKL on a PGC1α responsive promoter /reporter gene. The results indicated that HKL was capable of activating this promoter in the presence of Sirt3, and not when Sirt3 was absent, suggesting that HKL can activate Sirt3 expression via activating PGC1α-dependent Sirt3 gene transcription ( Fig. 9f ). To confirm these results, we took advantage of the HeLa cells that were stably transfected with Flag-SIRT3, where the expression of SIRT3 is under the control of a CMV promoter, and not under SIRT3 native promoter. These HeLa cells were treated with HKL, and its effect on the expression of SIRT3 was measured in the presence of a transcription inhibitor actinomycin D. No effect of HKL was observed on the expression levels of SIRT3 in the presence of actinomycin D, suggesting that conditions where no new mRNA was synthesized; HKL had no effect on the expression levels of SIRT3 ( Supplementary Fig. 10 ). As in this experiment SIRT3 expression was under the control of a CMV promoter, negative results of this experiment also indicated that HKL induces SIRT3 expression by activating its own gene promoter. These results thus suggests that HKL activates Sirt3 via binding to protein, and this in turn could activate PGC1α-responsive Sirt3 gene promoter leading to increased levels of Sirt3. In this study we report identification of a biphenolic compound, HKL, as an activator of Sirt3. HKL treatment attenuated the agonist-induced hypertrophic response of cardiomyocytes in vitro , as well as pressure overload cardiac hypertrophy in vivo . We also demonstrate that HKL is capable of blocking pre-existing cardiac hypertrophy in mice, a finding highly relevant to clinical cardiology. In addition, we show that HKL treatment prevents induction of cardiac fibrosis by attenuating fibroblast proliferation and transformation into myofibroblasts. To the best of our knowledge this is the first report describing an activator of Sirt3 capable of deacetylating mitochondrial targets and blocking cardiac hypertrophic response. Cardiomyocytes are densely packed with mitochondria to meet its high energy demand [35] . One of the consequences of this is the generation of ROS from mitochondria. These ROS at moderate levels are vital for cellular functions as they act as signalling molecules and activators of host defense by killing pathogens [36] . On the flipside, imbalance between ROS generation and its clearance by antioxidants results in oxidative stress and cellular damage. One of the antioxidants present in mitochondria is MnSOD. Recent studies have shown that MnSOD activity is post translationally modified by reversible lysine acetylation. Acetylation of MnSOD at lysine-122 decreases its activity [28] . The deacetylase responsible for its activation was found to be Sirt3 (refs 17 , 28 ). In the present study we found that HKL treatment increased Sirt3 levels, and this was associated with reduced acetylation of MnSOD. We also found increased acetylation of MnSOD in mice subjected to TAC, whereas treatment with HKL helped to maintain MnSOD deacetylation level similar to controls. Further, our results show that HKL could lower H 2 O 2 -induced ROS synthesis in the presence of Sirt3. This was associated with reduced H 2 O 2 -induced cell death of Sirt3 wild-type cells pretreated with HKL, but not Sirt3-KO cells. Sirt3 can also regulate mitochondrial function through several other mechanisms and is considered a major regulator of mitochondrial acetylome during calorie restriction, the most robust intervention to retard ageing [5] . In human liver, reversible acetylation is thought to regulate enzymes involved in glycolysis, gluconeogenesis, TCA cycle, urea cycle, fatty acid metabolism and glycogen metabolism, and the health of mitochondria can be assessed by measuring the oxygen consumption rate [37] , [38] . Sirt3-KO mice exhibit decreased oxygen consumption rate and develop oxidative stress [12] . In the same vein, overexpression of Sirt3 is associated with increased oxygen consumption rate and reduced oxidative stress [39] . Consistent with these observations, we found increased oxygen consumption in Sirt3 wild-type cells treated with HKL, but not in Sirt3-deficient cells. All these findings strongly suggest that the cellular effects of HKL could be mediated through activation of Sirt3. In the heart, overexpression of Sirt3 protects cardiomyocytes from death and hypertrophic stimuli [1] , [7] . Sirt3-deficient mice are susceptible to develop cardiac hypertrophy accompanied by fibrosis at an early age [1] , [40] . They also develop augmented cardiac hypertrophy in response to agonists, which can be blocked by overexpressing Sirt3 (ref. 1 ). Increased activation of Sirt3 activates MnSOD and reduces ROS levels, thereby suppressing Ras activation and downstream signalling through MAPK/ERK and PI3K/Akt pathways. Correspondingly, HKL has been shown to attenuate cancer cell progression by inactivating RAS or by activating the LKB1/AMPK pathway [41] . Consistent with this observation, previously, we have shown that Sirt3 also blocks ROS-mediated Ras activation and activates LKB1, thereby suppressing Akt signalling and activating AMPK in cardiomyocytes and protecting the heart from hypertrophic stimuli [1] , [42] . HKL also inhibits STAT3 in transformed Barrett’s cells, and can prevent phosphorylation of Akt and ERK2 (ref. 43 ). There are also reports showing that HKL suppresses MAPK signalling pathway by suppressing the phosphorylation of p38 mitogen-activated protein kinase (MAPK), extracellular signal-regulated kinase (ERK) and c-Jun N-terminal kinase (JNK) [44] . HKL was also shown to protect the rat brain against ischaemia-reperfusion injury and inhibited the HIF1α pathway, which is also reported to be negatively regulated by Sirt3 (refs 9 , 27 , 45 ). In lines with these observations, in the current study we found that Sirt3 activation by HKL blocks over activation of Akt and its downstream kinases, thus blocking development of cardiac hypertrophy. Because of these common effects, a possibility exists that many of the previously reported cellular effects of HKL could be explained via its ability to activate Sirt3. In this study, we also examined the effect of HKL on SIRT1 and found no change in expression levels of this sirtuin. SIRT1 is known to deacetylate and activate Akt in cardiomyocytes [46] . As we found opposite results, that is, suppression of Akt activity by HKL, the possibility of HKL activating SIRT1 enzymatic activity can be also excluded. Another important finding reported here is the ability of HKL to block cardiac fibrosis in a Sirt3-dependent manner. A role of Sirt3 in regulation of cardiac fibrosis has never been investigated. We found that treatment of cardiac fibroblasts with HKL resulted in a dose-dependent decrease in cardiac fibroblasts proliferation due to G0/G1 arrest without any appreciable toxicity, suggesting that the anti-proliferative effect of HKL is not due to its cytotoxic effects. Sirt3-KO fibroblasts spontaneously differentiate into myofibroblasts, and treatment with HKL has no effect on this transformation, whereas in wild-type cells HKL treatment attenuated the phenotypic transformation of fibroblasts into myofibroblasts, thus suggesting that Sirt3 is needed for anti-fibrotic effects of HKL. These results were confirmed in vivo , where mice treated with HKL developed significantly less fibrosis when subjected to aortic banding or isoproterenol infusion, compared with untreated mice. Conversely, HKL-treatment did not protect Sirt3-KO mice from developing cardiac hypertrophy and fibrosis. These results suggest that pharmacological activation of Sirt3 by HKL could be a potential therapeutic strategy to prevent adverse cardiac remodelling and other diseases associated with abnormal cellular growth and organ fibrosis. How does HKL activate Sirt3? Experiments carried out to understand the mechanism behind the ability of HKL to activate Sirt3 indicated that HKL physically binds to Sirt3. Correspondingly, we found that HKL can enter into mitochondria, suggesting that mitochondria could be the site of this interaction. Although we have not resolved the mechanism involved in the transportation of HKL to mitochondria, previous studies have reported that many hydrophobic compounds like HKL can enter into mitochondria simply by diffusion across the membrane [47] , [48] . The physical interaction of Sirt3 with HKL may enhance Sirt3’s deacetylase activity. We found that recombinant Sirt3 incubated with HKL had increased affinity for NAD. This increased Sirt3’s affinity for NAD could be critical in combating stress. We have previously shown that cardiac hypertrophy is associated with depletion of NAD, which could be resulting due to increased activity of NAD consuming enzymes such as PARP and CD38 (refs 42 , 49 ). Also NAD can be lost through the opening of hemichannels [50] , [51] . Direct activation of Sirt3 by HKL by increasing its affinity for NAD will help Sirt3 to remain active under pre-existing stress conditions. In agreement with this, we found that HKL treatment blocked pre-existing cardiac hypertrophy in mice. Activation of Sirt3 by HKL in the mitochondria can also replenish the lost NAD levels. NADH generated in the glyceraldehyde 3 phosphate dehydrogenase reactions can be deoxidized to NAD via the pyruvate dehydrogenase, the citric acid cycle and the mitochondrial respiratory chain [52] . Recent studies show that activities of enzymes involved in these pathways are regulated by reversible acetylation. Well-characterized substrates of Sirt3 include TCA cycle enzymes and enzymes that provide substrates for TCA cycle [53] . Sirt3 also deacetylates protein subunits in the electron transport chain and fatty acid oxidation [31] , [54] . These findings suggest that direct activation of Sirt3 by HKL can have immediate consequences on cell survival and growth. Besides post-translational activation, we found that HKL can also increase Sirt3 mRNA levels. Though we have not explored the mechanism for increased mRNA levels of Sirt3 in detail, as that was not the goal of this study, our results show that it could be achieved through PGC1α-dependent activation of Sirt3 gene transcription. It is reported that PGC1α increases the Sirt3 gene transcription through co-activation of the orphan nuclear receptor ERRα (oestrogen-related receptor alpha) [34] . Moreover, PGC1α levels are also downregulated in Sirt3-KO mice [18] . In this study we found that a PGC1α responsive promoter could be activated by HKL only in wild-type cells, and not in Sirt3-KO cells. These findings suggested that post-translational activation of Sirt3 leads to activation of Sirt3 gene promoter by a PGC1α-dependent mechanism, and therefore increased expression of Sirt3 mRNA levels. It is worth mentioning that PGC1α has been shown to be downregulated in hypertrophied and failing hearts, which is consistent with our observation of reduced Sirt3 levels in TAC-induced cardiac hypertrophy [55] , [56] , [57] . On the basis of data presented here and published before, we propose a model in Fig. 10 explaining the possible mechanism behind the activation of Sirt3 by HKL, and its ability to block cardiac hypertrophic response. Because Sirt3 regulates many aspects of mitochondrial function and oxidative stress is a prime cause for many diseases, we believe that HKL may prove to be beneficial in the management of wide variety of diseases. 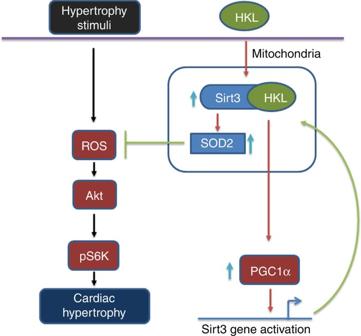Figure 10: Model illustrating the mechanism of Sirt3 activation by HKL. In cardiomyocytes HKL can directly bind to and activate Sirt3. Increased activity of Sirt3 promotes deacetylation of mitochondrial targets, including MnSOD. These reactions lead to reduced synthesis of ROS and thereby reduced cellular oxidative stress. Activated Sirt3 can also cause activation of PGC1α, which activatesSirt3gene promoter, leading to increased synthesis of Sirt3 mRNA transcripts. Increased activity of Sirt3 blocks cardiac hypertrophic response by suppressing ROS production and Akt activation, as reported by us before1. Figure 10: Model illustrating the mechanism of Sirt3 activation by HKL. In cardiomyocytes HKL can directly bind to and activate Sirt3. Increased activity of Sirt3 promotes deacetylation of mitochondrial targets, including MnSOD. These reactions lead to reduced synthesis of ROS and thereby reduced cellular oxidative stress. Activated Sirt3 can also cause activation of PGC1α, which activates Sirt3 gene promoter, leading to increased synthesis of Sirt3 mRNA transcripts. Increased activity of Sirt3 blocks cardiac hypertrophic response by suppressing ROS production and Akt activation, as reported by us before [1] . Full size image Primary cultures of cardiomyocytes Primary cultures of cardiac myocytes were prepared from neonatal rat hearts. In brief, hearts were removed from 1- to 3-day-old pups (Sprague-Dawley rats, either sex) and kept in cold DMEM. Ventricles were cut into 4 to 6 evenly sized pieces using small scissors and digested using collagenase type II (Worthington). The digested solution was collected with the cannula-syringe avoiding the tissue chunks and was added to one of the already aliquoted 10 ml FBS (100%). These steps were repeated six to seven times till no tissue chunks are visible. Tissue digest was spun and pellet was dissolved in DMEM with 5% FBS. Cells were pre-plated for 1 h to remove fibroblasts, and unattached cardiomyocytes in suspension were collected and plated in fibronectin-coated culture plates. Cardiomyocytes cultures were used after 24 h of plating. [ 3 H]Leucine incorporation Cardiomyocytes cultures were treated with PE (20 μM) or angiotensin-II (Ang, 0.1 μM) in the presence or absence of HKL. Immediately after treatment with agonists, cells were incubated with [ 3 H]-leucine (1.0 mCi ml −1 , 163 Ci mmol −1 specific activity, Amersham biosciences) (Invitrogen) for 24 h. Cells were washed with PBS and then incubated in 10% trichloro acetic acid to precipitate proteins. The resultant pellet was solubilized in 0.2 N NaOH and diluted with one-sixth volume of scintillation fluid, and the radioactivity was measured in a scintillation counter. Values were normalized with DNA content, which was measured by use of Quant-iT picogreen dsDNA assay kit (Invitrogen). Transfection/infection and luciferase assay For NFAT luciferase assay neonatal rat cardiomyocytes were infected with luciferase reporter vector containing multiple NFAT-binding sites. Twelve hours after infection cells were treated with PE (20 μM) or angiotensin-II (Ang, 0.1 μM) for 8 h in the presence or absence of HKL. HKL treatment was performed 2 h before agonist treatment. Luciferase activity assay was performed using the Luciferase activity assay kit from Promega, according to the manufacturer’s protocol. All transfections were performed using Lipofectamine 2000 (Invitrogen). BrdU assay Cell proliferation assay was performed using BrdU assay kit (BD Biosciences). In brief, neonatal rat cardiac fibroblasts cultured in complete growth medium were treated with 5 or 10 μM HKL. Sixteen hours after HKL treatment, cells were treated with BrdU (10 μM) for 2 h. Cells were harvested, stained with an anti-BrdU antibody and 7-AAD and subjected to FACS analysis. Antibodies The GAPDH antibody was purchased from Santa Cruz. The SIRT1 antibody was from Millipore and Nampt antibody was from Alexis. Ac-K 122 MnSOD and Ac-K 139 OSCP and OSCP antibodies were generated in Dr David Gius lab (Northwestern University). All other antibodies were purchased from Cell signaling. ROS detection ROS levels were detected using CM-H 2 DCFDA reagent (Invitrogen) as per the manufacturer’s instructions. In brief, primary cultures of cardiomyocytes were treated with H 2 O 2 (50 μM) in the presence or absence of HKL (10 μM) for 15 min. Cells were stained with CM-H 2 DCFDA. Cells were acquired by FACSCalibur and analysed with use of FlowJo. The mean fluorescence intensity of cells positive for CM-H 2 DCFDA staining was determined. Mitochondrial uptake of HKL Mitochondrial isolates were obtained from female WT mice using a differential centrifugation procedure modified from Savage et al , [32] and Roede et al , [58] Fresh liver was obtained immediately following euthanization with CO 2 , weighed and homogenized in 5 ml of incubation buffer (2 mg ml −1 bovine serum albumin, 220 mM mannitol, 70 mM sucrose, 2 mM HEPES and 1 mM EGTA) with 10 strokes from a dounce homogenizer. The homogenized tissue was centrifuged at 4 °C and 600 × g for 5 min. The supernatant was transferred to a new centrifuge tube and the pellet was re-homogenized, re-centrifuged and the remaining supernatant transferred. This suspension was then centrifuged at 4 °C and 11,000 × g for 11 min, upon which the supernatant was discarded and the pellet was re-suspended in fresh isolation buffer. Following an additional centrifugation at 600 × g for 5 min, the supernatant was added to a fresh tube and the mitochondria were pelleted at 8000 × g by centrifuging for 10 min. The resulting pellet was re-suspended in incubation buffer (250 mM sucrose, 10 mM MOPS, 3 mm KH 2 PO 4 , 5 mM succinate and 5 mM malate). The mitochondrial isolate, which is ∼ 90 pure with some contamination from lyosomes and peroxisomes, was assayed for total protein via bicinchoninic acid assay and viability by monitoring absorbance at 540 nm following dosing of 100 μg (as mitochondrial protein) with 15 μl of 2 mM CaCl 2 . HKL uptake within the freshly isolated mitochondria was determined at 0, 15 30 60 and 120 min by incubating mitochondria in a 10 μM HKL solution prepared in incubation buffer. HKL was first dissolved in EtOH to make a stock solution of 20 mM, which was then diluted 2,000:1 in chilled incubation buffer. For the HKL dosed and control isolates (0.05% EtOH in incubation buffer), 500 μg (400 μl total suspension volume) of mitochondrial protein was incubated on ice for the required time period, upon which the isolates were pelleted at 16,100 × g and 4 °C for 3 min, rinsed 3x with chilled incubation buffer, re-suspended in 150 μl LC-MS grade H 2 O, sonicated and stored at −80 °C until LC-HRMS analysis. Confirmation and quantification of HKL by LC-HRMS HKL was quantified within the dosed and controlled mitochondrial isolates via reverse phase chromatography and detection via a Q-Exactive high-resolution mass spectrometer operated in negative electrospray ionization mode (Thermo-Fisher, San Jose CA). Instrument operation parameters can be found in Roede, Uppal [58] . The m/z and retention time of HKL (265.1234 and 9.6 min, respectively) was confirmed using MS [2] analysis of the authentic reference standards. Mitochondrial isolates were prepared for analysis by adding 130 μl of LC-MS grade acetonitrile to 65 μl of mitochondria isolate. Following a 30-min incubation period, the sample extract was centrifuged at 16.1 × g and 4 °C for 10 min, and the supernatant was removed and analysed. Following LC-HRMS, data were extracted using apLCMS [59] with modifications by xMSanalyzer [60] . Quantification of HKL in the samples was determined by calculating the response factor (-H adduct, m/z =265.1229, 7.8 p.p.m. mass error) for a spiked mitochondrial isolate containing 1 μM HKL and multiplying by the averaged ion intensity for each time point following subtraction of the initial time point averaged intensity to account for irreversible binding. Mitochondrial swelling assay Rat liver mitochondria were isolated as described [61] . In brief, rats were anaesthetized with use of carbon-dioxide and killed by decapitation. Liver tissue (10–15 g) was removed and sliced in Buffer A ((EDTA–NaOH (pH 7) 0.1 mM, HEPES–KOH (pH 7.2) 10 mM, Leupeptin 1 μg ml −1 , Phenylmethanesulfonyl fluoride (PMSF)  0.15 μM, Sucrose 250 mM, final concentration)). Buffer A was added at a ratio of 3:1(v/w) and the liver was homogenized with a Teflon glass homogenizer. The homogenate was diluted 1:1 with buffer A and was centrifuged at 1,000 g for 5 min at 4 °C. Supernatant was collected and transferred to a new centrifuge tube and was centrifuged at 12,000 g for 10 min at 4 °C. Pellet was resuspended in 8 ml of buffer A/gram of pellet, and centrifuged at 12,000 g for 10 min at 4 °C. The resultant mitochondrial pellet was resuspended in buffer B ((HEPES–KOH (pH 7.2) 10 mM, Leupeptin 1 μg ml −1 , Phenylmethanesulfonyl fluoride (PMSF) 0.15 μM, Sucrose 250 mM, final concentration)). The isolated mitochondria were kept on ice and used within 2–4 h after preparation. Ca 2+ -induced large-amplitude mitochondrial swelling was assayed in freshly prepared mitochondria. The tested compound was added to mitochondria (0.5 mg ml −1 ), and CsA-sensitive mitochondrial swelling was initiated by the addition of Ca 2+ (0.1 mM) to the sample containing 0.2 mM Pi. Absorbance changes at 520 nm were monitored every 15–20 s with an Ultraspec 2100 spectrophotometer. Oxygen consumption rate measurement Cellular oxygen consumption rate of cardiac fibroblasts (12,000 cells/well) was determined using XF96 Seahorse system (Seahorse bioscience, Massachusetts) as per the manufacturer’s instructions. Real-time PCR analysis of mRNA levels Total RNA was isolated from mouse hearts by using Trizol Reagent (Invitrogen). The residual genomic DNA was digested by incubating the RNA preparation with 0.5 units of RNase-free Dnase-1 per microgram of RNA in 1 × reaction buffer for 15 min at room temperature, followed by heat inactivation at 90 °C for 5 min. The quality of DNase-1 treated RNA was tested by doing formaldehyde agarose gel electrophoresis. Two micrograms of DNase-treated RNA was reverse transcribed by use of Fermentas, RevertAid First Strand cDNA Synthesis Kit. The resultant cDNA was diluted 10-fold before PCR amplification. A reverse transcriptase minus reaction served as a negative control. The mRNA levels were measured by SYBR green real-time PCR. Primer sequences of genes used for RT-PCR analysis are given in Table 1 . Table 1 Sequences of primers used for RT-RCR analysis. Full size table Histology and immunohistochemistry For detection of cell size, frozen heart sections were stained with 10 μM wheat germ agglutinin coupled to tetramethylrhodamine isothiocynate (Sigma). Images were obtained using confocal microscopy. The cell size of myocytes was measured by use of NIH ImageJ software. Fibrosis was detected with use of Masson’s trichrome staining kit from Sigma, according to the manufacturer’s protocol. ANF release from nuclei of cardiomyocytes was determined by staining cells with antibodies specific for α-actinin and ANF. For determination of cell size, Image J software was used to calculate cardiomyocyte surface area of at least 50 cells (actinin-positive cells)/plate in an experimental group. Cardiomyocyte size was expressed as fold change with respect to untreated control. Imaging of cardiac fibroblasts Cardiac fibroblasts on 12-mm coverslips were treated with Ang or Ang plus HKL for 72 h. Cells were washed with PBS, and fixed with 3.7% formaldehyde in PBS for 15 min followed by permeabilization with 0.1% Triton X-100 for 5 min. It is then blocked with 10% BSA in PBS followed by incubation with primary antibody overnight at 4 °C. Thereafter, cells were incubated with a secondary antibody conjugated with either Alexa Fluor 594 or FITC for 1 h. Cells were washed and mounted in ProLong Gold antifade reagent with DAPI. Cells were visualized using a Leica SP2 laser scanning microscope. To quantify the myofibroblast transformation total fluorescence of each cell (100 cells in each group) were measured using the Image J software, and the results are presented as relative α-SMA, collagen or fibronectin levels. Induction of hypertrophy in mice The aortic banding was carried out in adult mice to produce pressure overload hypertrophy. Adult male CD-1 mice weighing ∼ 30 g (6–8 Weeks) were anaesthetized with ketamine (60 mg kg −1 , ip) and xylazine (10 mg kg −1 , ip) and ventilated with a small rodent ventilator (CWE, Ardmore, PA). The chest was opened by performing a ministernotomy, and the aorta was identified between the inominate and left common carotid arteries and dissected free from surrounding fatty tissue. A 4-0 ticron suture was tied around the aorta over a 26-gauge needle (28 guage where hypertrophy was established before HKL treatment) between the origin of the inominate and left common carotid arteries. In experiments the needle was subsequently removed. Adequacy of aortic constriction was demonstrated visually at this point by the difference between the bounding pulsations observed in the right common carotid artery (which arises from the inominate artery) and the near absence of visible pulsation in the left common carotid artery. Animals with sham surgery underwent an identical procedure with the exception of band placement. At the time of death, the presence of a band in the aorta was visually verified, and only those animals with an intact band in place were included in further study. For isoproterenol (ISO)-mediated cardiac hypertrophy, 8.7 mg kg −1 day −1 ISO was given for 7 days by implanting osmotic Minipumps (ALZET) into the abdomen of adult mice. HKL dissolved in peanut oil was injected at a rate of 0.2 mg kg −1 day −1 intraperitoneally. All animal protocols were reviewed and approved by the University of Chicago institutional animal care and use committee. Echocardiography of mice Chest hairs of mice were removed with a topical depilatory agent and transthoracic echocardiography was performed under inhaled isoflurane ( ∼ 1%) for anaesthesia, delivered via nose cone. Limb leads were attached for electrocardiogram gating, and the animals were imaged in the left lateral decubitus position with a VisualSonics Vevo 770 machine, using a 30 MHz high-frequency transducer. Body temperature was maintained using a heated imaging platform and warming lamps. Two-dimensional images were recorded in parasternal long- and short-axis projections, with guided M-mode recordings at the midventricular level in both views. LV (left ventricle) cavity size and wall thickness were measured in at least three beats from each projection and averaged. LV wall thickness (interventricular septum [IVS] and posterior wall [PW] thickness) and internal dimensions at diastole and systole (LVIDd and LVIDs, respectively) were measured. LV fractional shortening ([LVIDd—LVIDs]/LVIDd) and relative wall thickness ([IVS thickness+PW thickness]/LVIDd) were calculated from the M-mode measurements. Fluorescence anisotropy The steady-state fluorescence anisotropy measurements were performed with a Photon Technology Instruments (PTI) spectrofluorometer using a 1-cm path length quartz cuvettes at room temperature ( ∼ 23 °C). Excitation and emission slits with a band-pass of 2 nm were used for all measurements. The anisotropy values were calculated from the equation1 where I VV and I VH are the measured fluorescence intensities (after appropriate background subtraction) with the excitation polarizer vertically oriented and emission polarizer vertically and horizontally oriented, respectively. G is the instrumental correction factor and is the ratio of the efficiencies of the detection system for vertically and horizontally polarized light and is equal to I HV / I HH . Statistical analysis Statistical differences among groups were determined with either Student’s t -test (for two groups) or one-way analysis of variance (ANOVA). P values less than 0.05 was considered significant. How to cite this article : Pillai, V.B. et al , Honokiol blocks and reverses cardiac hypertrophy in mice by activating mitochondrial Sirt3. Nat. Commun , 6:6656 doi: 10.1038/ncomms7656 (2015).